A natural riboswitch scaffold with self-methylation activity Methylation is a prevalent post-transcriptional modification encountered in coding and non-coding RNA. For RNA methylation, cells use methyltransferases and small organic substances as methyl-group donors, such as S -adenosylmethionine (SAM). SAM and other nucleotide-derived cofactors are viewed as evolutionary leftovers from an RNA world, in which riboswitches have regulated, and ribozymes have catalyzed essential metabolic reactions. Here, we disclose the thus far unrecognized direct link between a present-day riboswitch and its inherent reactivity for site-specific methylation. The key is O 6 -methyl pre-queuosine (m 6 preQ 1 ), a potentially prebiotic nucleobase which is recognized by the native aptamer of a preQ 1 class I riboswitch. Upon binding, the transfer of the ligand’s methyl group to a specific cytidine occurs, installing 3-methylcytidine (m 3 C) in the RNA pocket under release of pre-queuosine (preQ 1 ). Our finding suggests that nucleic acid-mediated methylation is an ancient mechanism that has offered an early path for RNA epigenetics prior to the evolution of protein methyltransferases. Furthermore, our findings may pave the way for the development of riboswitch-descending methylation tools based on rational design as a powerful alternative to in vitro selection approaches. In recent years, numerous discoveries of metabolite-sensing riboswitches hint at RNA World ribozymes that could have promoted chemical transformations [1] , [2] , [3] . One hypothesis suggests that present-day riboswitches for common enzyme cofactors may have evolved from ancient ribozymes that depended on these cofactors [4] , [5] , [6] , [7] . What has stood the test of time are RNA sensors of cofactors for the regulation of gene expression [8] while the reactivity part has been taken over by more efficient protein-based modification machineries [9] , [10] , [11] , [12] . Riboswitches typically employ a highly conserved aptamer domain to sense the small molecule ligand with high specificity and selectivity, and an adjoining expression platform to regulate the expression of genes associated with ligand biosynthesis and transport [8] , [13] , [14] . Thereby, the partially overlapping RNA sequences of the two domains assist in converting the ligand-binding event into a change in gene expression by employing ligand-mediated RNA folding changes. It seems reasonable to assume that ligand-induced structural adaptions may also be exploited to trigger a chemical reaction. A single example exists for a known naturally occurring RNA, namely the glms riboswitch-ribozyme which binds glucosamine-6-phosphate whose protonated amino group then directly participates in reaction catalysis of RNA backbone cleavage [15] . Moreover, support for an advanced reactivity scope of cofactor-RNA systems has been provided by ribozyme engineering. The first methyltransferase ribozyme that catalyzes the site-specific installation of 1-methyladenosine in a substrate RNA, using a small-molecule cofactor has been created by in vitro evolution very recently [16] . Numerous natural riboswitches are known to selectively sense nucleotide-derived metabolites connected to methyl-group transfer or one-carbon metabolism, comprising SAM, methylene tetrahydrofolate (THF) and adenosylcobalamin (vitamin B12) [17] . The aptamers of these riboswitches bind their dedicated ligands in the nano- to micromolar range. For all of them, different subclasses are found, meaning that the ligand is recognized by distinct RNA architectures with both specific binding pockets as well as overall folds [18] . For SAM-binding riboswitches, a total of six subclasses is known to date; they accommodate the ligand with its reactive methyl group in conformations that strictly avoid self-methylation [19] , [20] . Therefore, it has remained an open question whether riboswitches can catalyze site-specific methylation reactions to produce defined methylated RNA products [9] , [11] . Besides the above-mentioned ubiquitous enzyme cofactors, other small organic compounds could serve for RNA-catalyzed RNA methylation in modern riboswitches, as implicated by the recently in vitro selected RNA methyltransferase that utilizes O 6 -methyl guanine [16] . An obvious link between guanine riboswitches and the near-cognate ligand O 6 -methyl guanine was tested even prior to the in vitro selected methyltransferase, however, methylation was not observed [21] . Nevertheless, we speculated that other riboswitches sensing guanine-type ligands may possess the inherent reactivity for methyl group transfer that we were searching for. Here, we report on the identification of a riboswitch motif that uses O 6 -methyl pre-queuosine (m 6 preQ 1 ) as a small-molecule methyl-group donor, catalyzing site-specific methylation of a cytosine at the N3-atom, resulting in RNA sequence-specific installation of 3-methylcytidine (m 3 C) (Fig. 1 ). Fig. 1: RNA methyltransferase activity. RNA sequence-specific installation of N3-methyl cytidine (m 3 C) using the small molecule m 6 preQ 1 as cofactor has been discovered and is described in this study. The direct link between a present-day riboswitch scaffold and RNA-catalyzed methylation is reported. Full size image Reactivity predictions for the preQ 1 riboswitch and ligand requirements We started our ambitious scheme to uncover RNA methylation activity with the analysis of ligand binding sites of various riboswitches and soon focused on preQ 1 class I riboswitches (Fig. 2a ) for which high-resolution crystal structures of both ligand-free and ligand-bound states were available (Fig. 2b, c ) [22] , [23] , [24] . This choice was also guided by our hypothesis that the methylated version of the cognate ligand preQ 1 , namely m 6 preQ 1 , might be an excellent candidate for methyl group donation since m 6 preQ 1 should retain the majority of interactions with the RNA as encountered in the genuine ligand-riboswitch system. Moreover, the principal reactivity of m 6 preQ 1 is expected to be comparable to m 6 G that serves as cofactor in the recently in vitro selected RNA methyltransferase [16] . Fig. 2: Analysis of preQ 1 -I riboswitch structures in the light of reactivity prediction. a Sequence and secondary structure of the Tt preQ 1 -I riboswitch (minimal aptamer motif in black). b Cartoon representation of the three-dimensional fold of the preQ 1 -bound aptamer (pdb code 3Q50; DOI: 10.2210/pdb3q50/pdb). c Stick representation of the ligand-free pocket revealing that A14 slides into the pocket and fills the space of preQ 1 while C15 flips out and becomes exposed (pdb code 3Q51; DOI: 10.2210/pdb3q51/pdb). d Stick representation of the preQ 1 -bound riboswitch pocket with crucial atom numbers annotated in black. e Chemical structures illustrating the hydrogen bond network of preQ 1 in the riboswitch pocket and the 2’-OH group of G11 that comes close the Hoogsteen face of preQ 1 . f Structure of a putative base pair between C15 (imino tautomer) and m 6 preQ 1 in the preQ 1 -I riboswitch pocket. Full size image Figure 2a shows the sequence and secondary structure of the 33 nt long aptamer of the Thermoanaerobacter tengcongensis ( Tt ) preQ 1 riboswitch which adopts an H-type pseudoknot structure exhibiting low nanomolar affinity for preQ 1 (Fig. 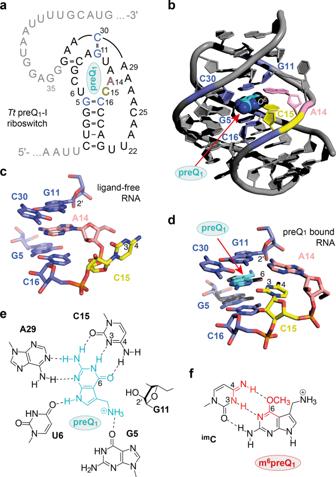Fig. 2: Analysis of preQ1-I riboswitch structures in the light of reactivity prediction. aSequence and secondary structure of theTtpreQ1-I riboswitch (minimal aptamer motif in black).bCartoon representation of the three-dimensional fold of the preQ1-bound aptamer (pdb code 3Q50; DOI: 10.2210/pdb3q50/pdb).cStick representation of the ligand-free pocket revealing that A14 slides into the pocket and fills the space of preQ1while C15 flips out and becomes exposed (pdb code 3Q51; DOI: 10.2210/pdb3q51/pdb).dStick representation of the preQ1-bound riboswitch pocket with crucial atom numbers annotated in black.eChemical structures illustrating the hydrogen bond network of preQ1in the riboswitch pocket and the 2’-OH group of G11 that comes close the Hoogsteen face of preQ1.fStructure of a putative base pair between C15 (imino tautomer) and m6preQ1in the preQ1-I riboswitch pocket. 2b ). The ligand is recognized by forming a Watson-Crick base pair with C15 (Fig. 2d,e ) while the ligand’s N3 hydrogen acceptor and the C2-NH 2 group are recognized in bidentate fashion via the Watson-Crick face of A29, complemented by a single H-bond between N9-H and the carbonyl oxygen of U6. Furthermore, a critical interaction responsible for the high affinity of preQ 1 is attributed to the 7-aminomethyl group and the carbonyl oxygen of G5. The tight binding pocket is further defined by preQ 1 stacking between the G5-C16 base pair and the nucleobase of G11 whose ribose 2′-OH is directed toward the preQ 1 O6 atom and the 7-aminomethyl group (Fig. 2e ). Importantly, the crystal structure of the ligand-free Tt RNA (Fig. 2c ) points at the high flexibility and structural dynamics of parts of the binding pocket: C15 is now directed outwards while the nucleobase of its next neighbor (A14) slides into the stacked position filling the space of the former C15-preQ 1 base pair. Because of the above-highlighted characteristics in structure and structural dynamics of the preQ 1 class I binding site we anticipated a high probability that the ligand congener m 6 preQ 1 transfers its methyl group to the RNA: First of all, recognition of m 6 preQ 1 by wild-type C15 should be easily possible if the tautomeric equilibrium is shifted towards the imino tautomer im C15 (Fig. 2f ). Second, the wild-type RNA pocket provides sufficient space to accommodate the methyl group (Fig. 2b,d ). Third, there are three potential nucleophilic groups for methylation available in the vicinity of the methyl group if m 6 preQ 1 becomes recognized by the pocket: these are the 2′-OH of G11, the C4-NH 2 of C15, and the N3 of C15 (Fig. 2 d,e ). Identification of methylated RNA product and reaction conditions A methylation product of the preQ 1 riboswitch would be difficult to distinguish from the unmodified RNA by gel shift or HPLC assays because its expected retention time will hardly differ. Therefore, we set out for an advanced mass spectrometric technology, Fourier-transform ion cyclotron resonance (FT-ICR) mass spectrometry (MS), which can determine the mass-to-charge ratio (m/z) of ions with very high precision by measuring the frequency of their cyclotron motion in a static magnetic field [25] , [26] . A major strength of such a set-up is that an RNA can be directly sequenced along with the identification of modifications and their localization (top-down RNA characterization) as we have demonstrated earlier [27] . We prepared the 33 nt long Tt preQ 1 riboswitch by RNA solid-phase synthesis, synthesized the m 6 preQ 1 ligand, and for initial trials, incubated both in a riboswitch-typical aqueous buffer system (2.5 µM RNA, 75 µM m 6 preQ 1 , 50 mM MOPS, 100 mM KCl, 2 mM MgCl 2 , pH 7.0). The reaction mixture was left overnight at room temperature, after which ultrafiltration with centrifugal concentrator devices was applied to remove the ligand and salts from the RNA for direct characterization by electrospray ionization (ESI) FT-ICR MS. Encouragingly, the high-resolution FT-ICR mass spectrum indeed showed the anticipated signal with a 14.0157 Da mass increase, consistent with a methyl group attached to the RNA (Fig. 3a ). The power of FT-ICR mass spectrometry is further manifested in the fact that backbone cleavage by collisionally activated dissociation (CAD) produced a complete set of c and y fragments (Fig. 3b,c ) that allowed for sequence determination (Fig. 3c ). The fragment mass values unequivocally revealed the site of methylation at the C15 nucleoside. Furthermore, the loss of methyl-C from RNA ions (Fig. 3d ) is direct evidence that the methyl group is located at the nucleobase. With respect to the precise position, the observed ratio for C to methyl-C of 3:1, which is higher than the statistical ratio of 8:1 according to the number of Cs in the sequence, suggests the N3 atom because methylation at the imino group generates a positive charge that weakens the glycosidic bond and in consequence facilitates base loss. Fig. 3: FT-ICR mass spectrometric characterization of the methylated RNA product. a ESI mass spectrum of the 33 nt m 3 C Tt preQ 1 -I RNA; the inset shows the isotopically resolved signal of the (M–10H) 10- ions; asterisks indicate piperidine RNA adducts. b Collisionally activated dissociation (CAD) of (M–nH) n– ions of RNA in the collision cell produces c and y fragment ions from RNA backbone cleavage. c Fragment-ion map illustrating sequence coverage from CAD of the methylated Tt preQ 1 -I RNA. The numbering of c and y fragments starts from the 5’ and 3’ terminus, respectively (top). MS signals of unmodified and methylated c 13 , c 14 , c 15 , c 16 , and complementary y 20 , y 19 , y 18 , y 17 fragments from CAD of (M−7H) 7− and (M–10H) 10− ions reveal the site of methylation (C15); the calculated isotopic profiles for unmodified and singly methylated RNA are indicated by red open circles. d Loss of methylated cytosine (red) in spectra from collisionally activated dissociation (CAD) of (M–10H) 10- ions of RNA is direct evidence for C nucleobase methylation; the 1:3 ratio of m 3 C/C nucleobase losses is consistent with destabilization of the glycosidic bond as a result of methylation at the N3 position. Full size image To be able to rapidly analyze the methylation reaction, we optimized anion-exchange HPLC conditions, resulting in clear baseline separation of the methylation product from the unmodified RNA (Fig. 4a ). We then tested different reaction conditions. Most importantly, when we decreased the pH from 7.0 to 6.0, the reaction yields increased to a significant extent, approaching 50% after 24 h which is the maximum yield possible, considering that the cognate preQ 1 ligand (with low nanomolar affinity) [21] , [28] released during the methylation reaction will be bound by the riboswitch/ribozyme, thereby blocking the binding of m 6 preQ 1 (Fig. 4b and Supplementary Fig. 1a ). We note that upon removal of the low molecular weight compounds by ultrafiltration, followed by adding a new batch of m 6 preQ 1 the reaction yields were increased further (Supplementary Fig. 1a ). Importantly, the reaction rate was dependent on m 6 preQ 1 concentration, with an apparent Michaelis constant K m of about 230 μM (Fig. 4c and Supplementary Fig. 1b ). In this context, we mention that when a one-fold excess of m 6 preQ 1 over RNA was applied only, methylation yields still amounted to 25% (Supplementary Fig. 1b ). Fig. 4: Reactivity scope of the Tt preQ 1 -I riboswitch scaffold. a Anion-exchange HPLC analysis of the preQ 1 -I RNA-catalyzed reaction with m 6 preQ 1 at 37 °C; 2.5 μM RNA substrate, 225 μM m 6 preQ 1 , 2.0 mM MgCl 2 , pH 6.0. HPLC traces of unmodified RNA, the reacted mixture, and the corresponding m 3 C-modified synthetic RNA reference is shown for comparison (for reaction time course see Supplementary Fig. 1b ). The m 3 C-modified RNA elutes earlier. Incubation of m 3 C preQ 1 -I RNA (isolated from a typical methylation reaction with m 6 preQ 1 ) under harsh basic conditions produced m 3 U from m 3 C under concomitant RNA hydrolysis (for FT-ICR MS characterization of m 3 U-RNA see Supplementary Fig. 1e ); chemical structures of m 3 C-to-m 3 U hydrolysis. b preQ 1 -I RNA reactivity analysis using diverse buffer conditions, nucleobase mutagenesis, atomic mutagenesis, and near-cognate cofactors; bars (gray) show mean ± s.e.m. ( n = 3 independent experiments); HPLC traces are depicted in Supplementary Fig. 2 , 3 ; source data are provided in the Source Data file. c The reaction rate is dependent on m 6 preQ 1 concentration. The observed rate constants k obs were determined based on HPLC trace analysis at five concentrations of m 6 preQ 1 , ranging from 25 to 300 μM. The red line represents a curve fit to k obs = k max [m 6 preQ 1 ]/( K m,app + [m 6 preQ 1 ]). Individual data points (open circles) ( n = 3 independent experiments), mean ± s.e.m. (black circles); source data are provided in the Source Data file. d Chemical structures for c 3 C and dG used in atomic mutagenesis reactivity assay. e Proposed reaction mechanism of preQ 1 -I RNA–catalyzed methylation using m 6 preQ 1 as cofactor; key features are the syn -conformation of the methyl iminoester moiety and N1 protonation of m 6 preQ 1 ; furthermore, coordination of the 2’-OH G11 to O 6 of m 6 preQ 1 assists in cofactor alignment and contributes to improve leaving group quality. f UV-spectroscopic determination of the p K a value of m 6 preQ 1 ( n = 3 independent experiments); source data are provided in the Source Data file. g Representative isotherm and ‘One set of sites’ binding­model fit for the preQ 1 class I riboswitch titrated with preQ 1 (left) and m 6 preQ 1 (right); the indicated K d values were determined at pH 6 ( n = 3 independent experiments); source data are provided in the Source Data file; one experiment for preQ 1 is depicted (left): N = 0.97, K A = 2.37 × 10 7 M −1 , Δ H = −27.57 × 10 3 cal mol ­1 , and Δ S = −58.7 cal (mol K) ­1 ; one experiment for m 6 preQ 1 is depicted (right): N = 0.99, K A = 1.36 × 10 4 M −1 , Δ H = −12.85 × 10 3 cal mol ­1 , and Δ S = −24.2 cal (mol K) ­1 . h Chemical structures of other potential cofactors tested. Full size image To unequivocally confirm the site of methylation, we synthesized m 3 C phosphoramidite for RNA solid-phase synthesis and prepared the corresponding m 3 C15 containing RNA reference (Fig. 4a ). This RNA had the same retention time as the product obtained by methylation using m 6 preQ 1 . We further point out that the synthetic m 4 C15 and m 5 C15 RNA references had retention times that were undistinguishable from the unmodified RNA in our HPLC assay (Supplementary Fig. 1c ). Therefore, we separated the m 3 C RNA product from a methylation reaction mixture and analyzed the remaining RNA by FT-ICR mass spectrometry, but no further methylation products were detected (Supplementary Fig. 1d ). Furthermore, we exposed the isolated m 3 C15 RNA to harsh basic conditions (pH 10) and observed the expected m 3 C-to-m 3 U conversion product (beside emerging fragments from RNA degradation) which additionally confirms that m 3 C15 RNA was formed selectively (Fig. 4a and Supplementary Fig. 1e ). RNA sequence requirements and reaction mechanism Next, we set out to investigate the Tt preQ 1 class I riboswitch sequence requirements for methyl group transfer. We observed no methylation products when C15 was mutated either to 3-deazacytidine (c 3 C), U, A, or G (Fig. 4b,d and Supplementary Fig. 2 ). In contrast, when C15 was mutated to 5-methylcytidine (C15m 5 C), methylation occurred almost as efficiently as for wildtype RNA (Fig. 4b and Supplementary Fig. 2 ). Furthermore, when the bulged-out nucleotide U12 close to the binding site, was deleted (mutant ΔU12), no methylation occurred (Fig. 4b ). U12, therefore, seems essential for retaining the structural dynamics within the U12-A13-A14-C15 segment. Moreover, when U6 and A29 which are crucial for recognition of the N9–N3 face of preQ 1 and m 6 preQ 1 were mutated individually to C and G, methylation was not observed anymore (Fig. 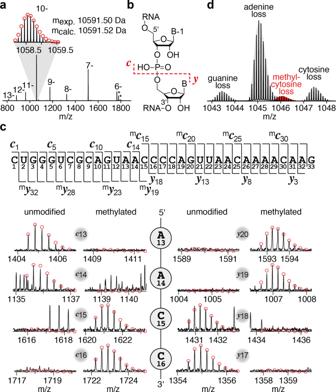Fig. 3: FT-ICR mass spectrometric characterization of the methylated RNA product. aESI mass spectrum of the 33 nt m3C Tt preQ1-I RNA; the inset shows the isotopically resolved signal of the (M–10H)10-ions; asterisks indicate piperidine RNA adducts.bCollisionally activated dissociation (CAD) of (M–nH)n–ions of RNA in the collision cell producescandyfragment ions from RNA backbone cleavage.cFragment-ion map illustrating sequence coverage from CAD of the methylatedTtpreQ1-I RNA. The numbering of c and y fragments starts from the 5’ and 3’ terminus, respectively (top). MS signals of unmodified and methylated c13, c14, c15, c16, and complementary y20, y19, y18, y17fragments from CAD of (M−7H)7−and (M–10H)10−ions reveal the site of methylation (C15); the calculated isotopic profiles for unmodified and singly methylated RNA are indicated by red open circles.dLoss of methylated cytosine (red) in spectra from collisionally activated dissociation (CAD) of (M–10H)10-ions of RNA is direct evidence for C nucleobase methylation; the 1:3 ratio of m3C/C nucleobase losses is consistent with destabilization of the glycosidic bond as a result of methylation at the N3 position. 4b and Supplementary Fig. 2 ). Importantly, compensatory mutation of the conserved base pair G5-C16 into C5-G16 gave a sevenfold decrease in yields for the m 3 C-modified RNA (Fig. 4b ), consistent with the crucial interaction of the O 6 -G5 atom and the protonated 7-aminomethyl group of preQ 1 or m 6 preQ 1 . Strikingly, we found evidence for a potential role of the 2′-OH group of G11 in the methyl transfer reaction. When we deleted this functional group (dG11 mutant), reaction yields decreased to one-fourth compared to the wild-type RNA (Fig. 4b,d ). This finding together with the above-described pH dependence of the reaction leads to the proposed reaction mechanism depicted in Fig. 4e . The favorable, slightly acidic pH value of 5–6 is consistent with saturating protonation of the 7-aminomethyl group and its recognition by G5. Importantly, it is also consistent with protonation of N1 of m 6 preQ 1 , thereby facilitating stabilization of the preQ 1 leaving group (Fig. 4f ). Our observation that methylation activity becomes impaired at pH values lower than 5 suggests protonation of N3 of C15, and hence the loss of nucleophilicity needed for an attack at m 6 preQ 1 . Furthermore, the model is compatible with stabilization of the syn conformation of the methyl iminoester by a hydrogen bond between m 6 preQ 1 O 6 and the 2′-OH of G11. Finally, we set out to estimate the affinity of m 6 preQ 1 to the riboswitch. Using isothermal titration calorimetry (ITC), we first determined the dissociation constant of the cognate preQ 1 ligand to wildtype preQ 1 RNA at pH 6 as reference (Fig. 4g ). The K d ITC value amounted to 43.0 ± 1.9 nM. We then determined the affinity of m 6 preQ 1 to the unreactive C15U RNA mutant and obtained a K d ITC value of 72.2 ± 2.1 µM at pH 6.0. This micromolar K d likely reflects the portion of pairing strength that arises from the identical recognition of the C7-CH 2 NH 2 moieties and the N9–N3–C2-NH 2 faces of preQ 1 and m 6 preQ 1 , respectively, by the pocket through A29 and U6. We note that A29G and U6C mutants were both inactive (Supplementary Fig. 2 ). Further, we believe that the actual affinity of m 6 preQ 1 to wild-type (C15) RNA is higher than to the unreactive C15U mutant because the imino tautomer im C15 as proposed in Fig. 2f could in principle provide a better match with respect to hydrogen donor-acceptor interactions compared to U15. Near-cognate cofactors and other preQ 1 riboswitch scaffolds Encouraged by our finding that a simple, methylated nucleobase can act as cofactor for riboswitch methylation, we set out to synthesize and test structural congeners of m 6 preQ 1 , namely O 6 -ethyl-preQ 1 (e 6 preQ 1 ), O 6 -benzyl-preQ 1 (bn 6 preQ 1 ), and O 6 -methyl-preQ 0 (m 6 preQ o ) (Fig. 4h and Supplementary Fig. 3 ). These derivatives, however, exhibited only very minor—or no—alkylation activities under optimized conditions (Fig. 4b and Supplementary Fig. 1f,g and Supplementary Fig. 3 ). Of further note, O 6 -methylguanine (m 6 G) and O 6 -(4-aminomethyl)benzylguanine (abn 6 G) did not result in detectable amounts of m 3 C15 RNA product (Fig. 4b ). The observation that the potential methyl group donors m 6 G and m 6 preQ 0 did not transfer their methyl groups can be rationalized by considering the significantly lower affinities of their non-methylated precursors, preQ 0 (17-fold lower) [22] and G (at least 25-fold lower) [29] compared to the cognate ligand preQ 1 . Therefore, it is reasonable to assume that m 6 preQ 1 is also significantly stronger bound compared to m 6 G and m 6 preQ 0 . It is the 7-aminomethyl substituent of preQ 1 and m 6 preQ 1 that has to be present together with its interaction partner, the G5-C16 base pair to reach high affinities [22] and high methylation yields (see G5C-C16G mutant, Fig. 4b ). We further note that e 6 preQ 1 and bn 6 preQ 1 which provide the 7-aminomethyl substituent exhibit lower yields likely because of steric hindrance of their larger O 6 substituents with the binding pocket. Next, we were wondering if representatives of the other known preQ 1 riboswitch classes also possess self-methylation properties [29] . Both, preQ 1 class II and III riboswitches have an identical architecture of their preQ 1 -bound pockets, however, this pocket architecture is different from class I [30] , [31] . Characteristically, class II and III apply a preQ 1 –C trans base pair instead of a cis Watson–Crick pair (class I), and significantly, the O 6 atom of preQ 1 is rather solvent-exposed with no obvious RNA functionalities for nucleophilic attack nearby. Nevertheless, we tested the well-studied preQ 1 II riboswitch from Lactobacillus rhamnosus for methyl transfer of m 6 preQ 1 ; as expected, methylation was not observed (Fig. 4b ). Noteworthily, class I preQ 1 riboswitches are categorized into three subtypes, with the Tt riboswitch belonging to type 1 [29] . We, therefore, complemented our analysis of RNA sequence requirements with a type 2 ( Bacillus subtilis ) and a type 3 preQ 1 riboswitch ( Shigella dysenteriae ). Both revealed no methyltransferase activity (Fig. 4b ). Our study answers the long-standing question of whether contemporary riboswitches can act as cofactor-dependent ribozymes by a clear yes. Direct evidence became possible after careful analysis of three-dimensional riboswitch architectures in combination with rational ligand design and chemical intuition that finally led to the discovery of methyltransferase activity of the Tt preQ 1 class I riboswitch. PreQ 1 itself is a guanine-derived precursor of the nucleobase queuosine (Q) that is found in the wobble position of tRNAs containing the GUN anticodon [32] . The presence of Q in tRNAs improves their ability to read degenerate codons, while the absence of enzymes participating in Q biosynthesis or salvage results in deleterious phenotypes in many organisms [33] , [34] . Noteworthily, O 6 -methylated versions of the pre-queuosine heterocycle have been found in nature, in form of 2-amino-5-cyano-4-methoxypyrrolo[2,3-d]pyrimidine produced by Streptomyces [35] , and as the corresponding N 2 -glyosylated natural products huimycin and dapiramicin [36] . Their occurrence hints at potential cellular availability of the near-cognate ligand m 6 preQ 1 for preQ 1 riboswitches. In this context it is also interesting that preQ 1 and SAM aptamers have been found in a putative tandem riboswitch architecture which might hint at the regulatory utility of linking m 6 preQ 1 biosynthesis to the concentrations of SAM and preQ 1 [29] , [35] , [36] . At this time, one can only speculate about the biological relevance of a riboswitch with potential self-methylation activity. Such a scenario implies that m 3 C methylation in the riboswitch pocket impairs recognition of the cognate ligand preQ 1 and thereby impacts the gene regulatory function of the riboswitch. 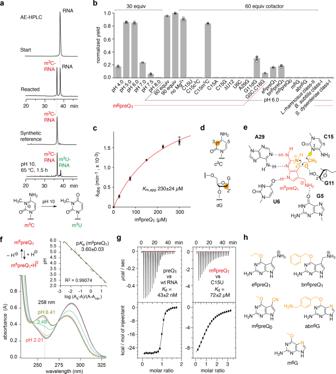Fig. 4: Reactivity scope of theTtpreQ1-I riboswitch scaffold. aAnion-exchange HPLC analysis of the preQ1-I RNA-catalyzed reaction with m6preQ1at 37 °C; 2.5 μM RNA substrate, 225 μM m6preQ1, 2.0 mM MgCl2, pH 6.0. HPLC traces of unmodified RNA, the reacted mixture, and the corresponding m3C-modified synthetic RNA reference is shown for comparison (for reaction time course see Supplementary Fig.1b). The m3C-modified RNA elutes earlier. Incubation of m3C preQ1-I RNA (isolated from a typical methylation reaction with m6preQ1) under harsh basic conditions produced m3U from m3C under concomitant RNA hydrolysis (for FT-ICR MS characterization of m3U-RNA see Supplementary Fig.1e); chemical structures of m3C-to-m3U hydrolysis.bpreQ1-I RNA reactivity analysis using diverse buffer conditions, nucleobase mutagenesis, atomic mutagenesis, and near-cognate cofactors; bars (gray) show mean ± s.e.m. (n= 3 independent experiments); HPLC traces are depicted in Supplementary Fig.2,3; source data are provided in the Source Data file.cThe reaction rate is dependent on m6preQ1concentration. The observed rate constantskobswere determined based on HPLC trace analysis at five concentrations of m6preQ1, ranging from 25 to 300 μM. The red line represents a curve fit tokobs=kmax[m6preQ1]/(Km,app+ [m6preQ1]). Individual data points (open circles) (n= 3 independent experiments), mean ± s.e.m. (black circles); source data are provided in the Source Data file.dChemical structures for c3C and dG used in atomic mutagenesis reactivity assay.eProposed reaction mechanism of preQ1-I RNA–catalyzed methylation using m6preQ1as cofactor; key features are thesyn-conformation of the methyl iminoester moiety and N1 protonation of m6preQ1; furthermore, coordination of the 2’-OH G11 toO6of m6preQ1assists in cofactor alignment and contributes to improve leaving group quality.fUV-spectroscopic determination of the pKavalue of m6preQ1(n= 3 independent experiments); source data are provided in the Source Data file.gRepresentative isotherm and ‘One set of sites’ binding­model fit for the preQ1class I riboswitch titrated with preQ1(left) and m6preQ1(right); the indicatedKdvalues were determined at pH 6 (n= 3 independent experiments); source data are provided in theSource Datafile; one experiment for preQ1is depicted (left):N= 0.97,KA= 2.37 × 107M−1, ΔH= −27.57 × 103cal mol­1, and ΔS= −58.7 cal (mol K)­1; one experiment for m6preQ1is depicted (right):N= 0.99,KA= 1.36 × 104M−1, ΔH= −12.85 × 103cal mol­1, and ΔS= −24.2 cal (mol K)­1.hChemical structures of other potential cofactors tested. 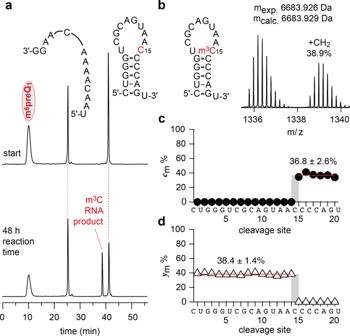Fig. 5: Methyltransferase activity using a split aptamer of preQ1-I RNA. aSequences of the twoTtpreQ1-I fragments used and anion-exchange HPLC traces of the reaction mixture at time points 0 and 48 h (25 μM each RNA strand, 1.5 mM m6preQ1, 2.0 mM MgCl2, 100 mM KCl, MES buffer pH 6.0, 37 °C); as expected, the m3C-modified RNA product elutes earlier.bSecondary structure of the m3C-modified preQ1-stem-loop RNA and CAD-MS of co-isolated (M − 5H)5-ions of unreacted 21 nt RNA (61.1%,mexp.6683.926 Da,mcalc.6683.929 Da) and methylated RNA (38.9%,mexp.6697.942,mcalc.6697.945 Da) produced at 65 eV laboratory frame energycandyfragments with and without methylation.cThereby, the fraction of methylatedcfragments (cm) increased from 0% to 36.8 ± 2.6% at site 15 (mean of values for sites 15 to 20 ± standard deviation).dThe fraction of methylatedyfragments (ym) decreased from 38.4 ± 1.4% to 0% at site 15 (mean of values for sites 1 to 14 ± standard deviation), which both are consistent with C15 as methylation site and with the yields independently obtained by HPLC analysis. Source data are provided in theSource Datafile. Thus far, the m 3 C modification itself is known for tRNAs in position 32 in diverse organisms [37] , [38] , ranging from yeast [39] , S. Pombe [40] , parasites such as Trypanosoma brucei [41] , to mice, rat, and human [42] . The modification has attracted additional interest when m 3 C has been identified as dynamic modification also in mRNA, and corresponding writer (METTL2, METTL6, METTL8) and eraser enzymes (ALKBH1, ALKBH3) have been characterized [43] . The emerging importance of the modification stimulated the development of novel RNA sequencing approaches, AlkAniline-Seq [44] and HAC-seq [45] , respectively, to reveal m 3 C sites transcriptome-wide. We furthermore anticipate that the discovered methyltransferase activity of the preQ 1 class I riboswitch can serve as starting point for engineering in vitro and in vivo methylation tools. Applications for m 3 C installation are conceivable not only in cis, but also in trans. First experimental attempts towards this aim by splitting the aptamer into two halves have been successful and led to remarkable 38% of methylation for the preQ 1 stem-loop by simply adding the 3′-terminal preQ 1 RNA fragment in the presence of cofactor (Fig. 5 ). Beyond methyltransferase activity and the particular m 3 C modification investigated here, our work may stimulate the search for other ribozyme-catalyzed reactions that are lying dormant in present-day riboswitches. Given the large number and great diversity of riboswitches that have been identified to date, a broad repertoire of chemical reactivities should be directly retrievable without the need for nucleic acids evolution that builds on constructed RNA libraries of naturally occurring riboswitch scaffolds [46] or on de novo in vitro RNA selection approaches [47] . Fig. 5: Methyltransferase activity using a split aptamer of preQ 1 -I RNA. a Sequences of the two Tt preQ 1 -I fragments used and anion-exchange HPLC traces of the reaction mixture at time points 0 and 48 h (25 μM each RNA strand, 1.5 mM m 6 preQ 1 , 2.0 mM MgCl 2 , 100 mM KCl, MES buffer pH 6.0, 37 °C); as expected, the m 3 C-modified RNA product elutes earlier. b Secondary structure of the m 3 C-modified preQ 1 -stem-loop RNA and CAD-MS of co-isolated (M − 5H) 5- ions of unreacted 21 nt RNA (61.1%, m exp. 6683.926 Da, m calc. 6683.929 Da) and methylated RNA (38.9%, m exp. 6697.942, m calc. 6697.945 Da) produced at 65 eV laboratory frame energy c and y fragments with and without methylation. c Thereby, the fraction of methylated c fragments ( c m ) increased from 0% to 36.8 ± 2.6% at site 15 (mean of values for sites 15 to 20 ± standard deviation). d The fraction of methylated y fragments ( y m ) decreased from 38.4 ± 1.4% to 0% at site 15 (mean of values for sites 1 to 14 ± standard deviation), which both are consistent with C15 as methylation site and with the yields independently obtained by HPLC analysis. Source data are provided in the Source Data file. Full size image Finally, we stress the importance of our findings for the RNA world hypothesis which postulates that possible early life on Earth relied on catalytic RNA properties essential for evolving sophisticated RNA-based life [5] , [6] , [7] , [8] , [9] , [10] , [48] . 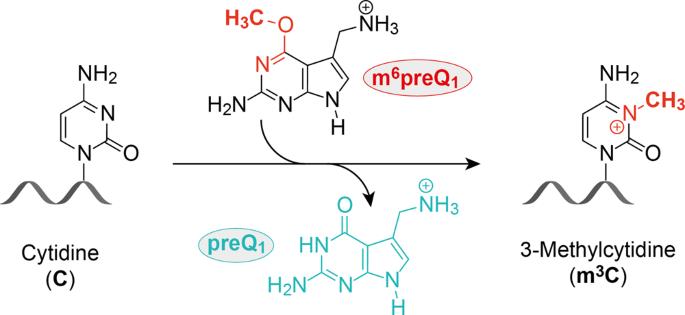The idea is strongly supported by the original discovery of bacterial riboswitches that regulate—without the aid of proteins—the expression of genes that are involved in the biosynthesis of metabolites [6] . Some of these riboswitches may have evolved from ancient cofactor-dependent ribozymes preserving their regulatory capacity while the reactivity part has been taken over by more efficient protein enzyme machineries. Our findings may also hint at a prebiotic version of RNA epigenetics with methylated nucleobases taking the role as cofactors for ancient methyltransferase ribozymes [49] , [50] , [51] , [52] . RNA synthesis RNA oligonucleotides were prepared by solid-phase synthesis using phosphoramidite chemistry (2′- O -TOM-protected) on controlled-pore glass solid supports [53] . Fig. 1: RNA methyltransferase activity. RNA sequence-specific installation of N3-methyl cytidine (m3C) using the small molecule m6preQ1as cofactor has been discovered and is described in this study. The direct link between a present-day riboswitch scaffold and RNA-catalyzed methylation is reported. RNA sequences are given in Supplementary Table 1 . Modified phosphoramidites for atomic mutagenesis and reference oligonucleotides were purchased (ChemGenes, Glen Research, Berry Asscociates) or prepared in-house, following published procedures [54] , [55] . RNA oligonucleotides were deprotected with ammonia and butylamine instead of ammonia and methylamine to avoid any possible methylated RNA from deprotection, followed by 1 M tetrabutylammonium fluoride in THF, desalted (Sephadex G25), and purified by denaturing anion exchange chromatography (Dionex DNAPac PA100, 9 × 250 mm, at 80 °C; solvent A was 25 mM Tris-HCl (pH 8.0) and 20 mM NaClO 4 in 20% aqueous acetonitrile; solvent B was 25 mM Tris-HCl (pH 8.0) and 0.6 M NaClO 4 in 20% aqueous acetonitrile; the gradient was: linear, 25–40% (25–45 for longer sequences) with slope of 5 % solvent B per column volume). Customized deprotection conditions were used for m 3 C RNA (3:1 (v/v) 28–30% aqueous NH 3 and EtOH, at 40 °C for 5 h), m 4 C RNA (O 4 -chlorophenyl U convertible nucleoside approach, 7 M NH 3 in MeOH at 42 °C for 18 h). The quality of RNAs (purity and identity) was analyzed by anion-exchange HPLC (Dionex DNAPac PA100, 2 × 250 mm, eluents as above, the gradient was: linear, 22–35% solvent B, with slope of 0.87% solvent B per column volume), and HR–ESI–MS (Thermo Fisher Orbitrap, negative-mode) or FT ICR MS (see below). Measured and calculated masses are listed in Supplementary Table 1 . Characterization of m 6 preQ 1 , e 6 preQ 1 , and bn 6 preQ 1 Analytical data (NMR spectra) of m 6 preQ 1 , e 6 preQ 1 , and bn 6 preQ 1 are shown in Supplementary Figs. 4 – 11 . m 6 G and abn 6 G were purchased from commercial sources (Carbosynth). Reaction of preQ 1 RNA with m 6 preQ 1 or analogs A typical methylation reaction was carried out in a volume of 200 μl containing 0.5 nmol RNA (2.5 µM) and 75 μM ligand (30 equiv) in buffer solution (2 mM MgCl 2 , 100 mM KCl, 50 mM 2-( N -morpholino) ethanesulfonic acid (MES), pH 6.0). After heating the mixture to 90 °C for 2 min, it was incubated for 48 h at 37 °C. After desalting using a Sep-Pak C18 cartridge, the methylated RNA product was directly analyzed in the mixture or isolated by AE HPLC, desalted again (Sep-Pak C18), and subjected to FT ICR-ESI-MS (which included a further desalting step using centrifugal concentrators; see below). For experiments at pH 4 and 5, sodium acetate buffer was used instead of MES; for pH 7, 7.5, and 8, MOPS was used. Several of the experiments were additionally analyzed using 60 and 120 equiv of the cofactor. The hydrolysis of m 3 C to m 3 U RNA was examined in a volume of 280 μl with 7 nmol RNA (25 µM) in 25 mM Na 2 CO 3 buffer (pH 10) with 1 mM EDTA at 65 °C for 1.5 h. After desalting (Sep-Pak C18) the m 3 U RNA was isolated by AE HPLC and analyzed by FT ICR–ESI–MS (see below). FT-ICR mass spectrometric analysis of RNA methylation/alkylation products Methanol was HPLC grade (Acros), ammonium acetate (≥99.0%, Na ≤5 mg/kg, K ≤ 5 mg/kg), piperidine (≥99.5%), and imidazole (≥99.5%, Na ≤ 50 mg/kg, K ≤ 50 mg/kg) were from Sigma-Aldrich, and H 2 O was purified to 18 MΩ·cm at room temperature using a Milli-Q system (Millipore). Experiments were performed on a 7T Fourier transform ion cyclotron resonance (FT-ICR) mass spectrometer (Bruker APEX ultra) equipped with an ESI source for (M − n H) n− ion generation and a collision cell through which a flow of Ar gas was maintained for CAD. The mass resolving power of this instrument is routinely (broadband detection, 2 M data points for a ∼ 2 s transient) ∼ 220,000, ∼ 120,000, and ∼ 80 000 at m / z 500, 1000, and 1500, respectively, and the mass accuracy is ∼ 1 ppm with internal calibration and ∼ 20 ppm with external calibration (Supplementary Table 1 ). RNA was electrosprayed (flow rate 1.5 µl/min) from 1–2 µM solutions in 1:1 or 9:1 H 2 O/CH 3 OH vol/vol with piperidine (2–10 mM) and imidazole (0–10 mM) as additives. Prior to dissociation by CAD, the (M − n H) n− ions under study were isolated in a linear quadrupole; for a more detailed description of the experimental setup for CAD see [56] . For statistical reasons, between 25 and 500 scans were added for each spectrum (20–50 for ESI, 100–500 for CAD), and data reduction utilized the SNAP2 algorithm (Bruker). For desalting, 400 µl of an ammonium salt solution (100 mM ammonium acetate in H 2 O) was added to 100 µl RNA solution (about 1 nmol in H 2 O) and concentrated to 100 µl using Vivaspin 500 centrifugal concentrators (Sartorius, MWCO 3000). The process was repeated five to seven times, followed by six to seven cycles of concentration and dilution with H 2 O. RNA concentration was determined by UV absorption at 260 nm using a NanoPhotometer (Implen). Kinetic assays of RNA-catalyzed methylation reactions The methylation reactions were carried out as described above (on a 1.5 nmol scale; 600 µl reaction volume) and 50-μl aliquots were taken at desired time points and quenched immediately by adding 50 μl of stop solution (12 M urea). The samples were analyzed by AE HPLC and UV-detection. The peak areas were quantified. The yield versus time data were fit to (fraction unreacted) = Y (1 − e – k t ), in which k = k obs and Y = final yield, using OriginPro (2020). All kinetic assays were carried out as three independent replicates. Isothermal titration calorimetry (ITC) ITC measurements were performed on a MicroCal iTC 200 instrument at 20 °C in 50 mM MES, 100 mM KCl and 2 mM MgCl 2 (pH 6.0). For preQ 1 , the concentration of Tte preQ 1 class I RNA in the measuring cell was typically 0.012 mM; preQ 1 ligand was in the syringe at a concentration that was 10-fold higher than the RNA. The c-value was typically around 300. For m 6 preQ 1 , the concentration of the Tte preQ 1 class I RNA in the measuring cell was typically 0.19 mM; m 6 preQ 1 cofactor was in the syringe at a concentration that was 15-fold higher than the RNA. The c -value was typically around 3. Both K d determinations were carried out as three independent replicates. Reporting summary Further information on research design is available in the Nature Research Reporting Summary linked to this article.